Controllable chirality-induced geometrical Hall effect in a frustrated highly correlated metal A current of electrons traversing a landscape of localized spins possessing non-coplanar magnetic order gains a geometrical (Berry) phase, which can lead to a Hall voltage independent of the spin–orbit coupling within the material—a geometrical Hall effect. Here we show that the highly correlated metal UCu 5 possesses an unusually large controllable geometrical Hall effect at T <1.2 K due to its frustration-induced magnetic order. The magnitude of the Hall response exceeds 20% of the ν =1 quantum Hall effect per atomic layer, which translates into an effective magnetic field of several hundred Tesla acting on the electrons. The existence of such a large geometric Hall response in UCu 5 opens a new field of enquiry into the importance of the role of frustration in highly correlated electron materials. Frustration is prevalent in nature, appearing in substances as simple as water ice to systems as complex as neural networks [1] , [2] . In general, frustration is the result of competing interactions of comparable strengths that can prevent a system from entering a single macroscopic lowest-energy configuration. The geometry of certain material structures is particularly prone to frustration, with the resulting degenerate ground states or near-ground states being highly susceptible to small perturbations and the emergence of exotic states of matter [1] , [2] . For example, frustration imposed by the geometrical arrangement of magnetic moments in electrical insulators induces novel states, such as spin-liquid, multiferroicity and magnetic monopole excitations in spin ice [1] , [2] , [3] , [4] , [5] , [6] , [7] . The absence of itinerant charge and spin degrees of freedom in magnetically frustrated insulators simplifies theoretical modelling of the microscopic origin and consequences of that frustration, and consequently, most studies have focussed on non-metallic materials. Nevertheless, geometrical frustration of spin configurations also may have significant consequences for metals, especially in highly correlated materials with itinerant electrons strongly coupled to localized spins [8] . One of those possible consequences is the emergence of a highly tunable and very large response of itinerant charge carriers to an applied magnetic field. In an ordinary metal, a Hall voltage V Hall arises perpendicular to both the current I and applied magnetic field H , and is related to the transverse resistivity ρ xy = V Hall /I = R 0 H , where R 0 is the Hall coefficient [9] . For a magnetic metal, however, scattering of itinerant electrons off of localized spins can produce additional contributions to ρ xy , typically proportional to the magnetization M and powers of the longitudinal resistivity ρ xx = V xx /I , resulting in so-called anomalous Hall effects described by Karplus and Luttinger [10] and skew-scattering theories [9] that are discussed in the Supplementary Methods section in the Supplementary Information . In addition, if frustration were to induce spin order in a non-coplanar structure, then itinerant electrons traversing the spin texture with local spin chirality ( Fig. 1a ) accumulate a chirality-induced Berry phase that also contributes to V Hall (refs 9 , 11 , 12 , 13 ). Theoretically, the effect of the spin texture on the current can reach the equivalent of a local magnetic field of H~ 10 4–5 T, which is at least two orders of magnitude larger than the highest field currently generated in high magnetic-field laboratories. Furthermore, if this local effective field does not average to zero over the sample, then the predicted Hall response can be as large as the integer quantum Hall effect in every atomic plane [14] , [15] , [16] , [17] . As the local spin chirality leading to such a large effective magnetic field and associated Hall response can be tuned by applying a much smaller external field, a clean example of such an effect would open a new direction towards designing functional materials with exotic properties and states. 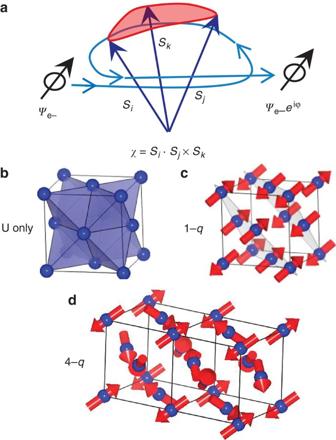Figure 1: Effect of spin chirality on an itinerant electron and UCu5's anti-ferromagnetic order. (a) A diagram illustrating the geometrical (Berry) phaseΦgained by an itinerant electron's wave function traversing the three non-coplanar spinsSi,SjandSkpossessing finite scalar spin chiralityχ.Ψe−is the incident wave function of the electron. (b) Illustration of the U sublattice of edge-sharing tetrahedra. (c) Illustration of the 1−qtype magnetic order whereq=<1/2,1/2,1,2>. (d) Illustration of the 4−qtype of magnetic order whereq=<1/2,1/2,1,2> For the 1−qorder, spins (red arrows) lie along [111], are ferromagnetically aligned within [111] planes, and anti-ferromagnetically aligned between them; whereas, the 4−qmagnetic order is non-coplanar, with spins pointing along various <111> directions with four propagation vectors:q=[1/2,1/2,1,2], [−1/2,1/2,1,2], [1/2,-1/2,1,2] and [1/2,1/2,-1,2]. For the 4−qorder, an electron traversing the non-coplanar spins acquires a chirality-induced Berry phase due to the mechanism shown ina. Illustrations inb,canddwere made using VESTA34. Figure 1: Effect of spin chirality on an itinerant electron and UCu 5 's anti-ferromagnetic order. ( a ) A diagram illustrating the geometrical (Berry) phase Φ gained by an itinerant electron's wave function traversing the three non-coplanar spins S i , S j and S k possessing finite scalar spin chirality χ . Ψ e− is the incident wave function of the electron. ( b ) Illustration of the U sublattice of edge-sharing tetrahedra. ( c ) Illustration of the 1− q type magnetic order where q =<1/2,1/2,1,2>. ( d ) Illustration of the 4− q type of magnetic order where q =<1/2,1/2,1,2> For the 1− q order, spins (red arrows) lie along [111], are ferromagnetically aligned within [111] planes, and anti-ferromagnetically aligned between them; whereas, the 4− q magnetic order is non-coplanar, with spins pointing along various <111> directions with four propagation vectors: q =[1/2,1/2,1,2], [−1/2,1/2,1,2], [1/2,-1/2,1,2] and [1/2,1/2,-1,2]. For the 4− q order, an electron traversing the non-coplanar spins acquires a chirality-induced Berry phase due to the mechanism shown in a . Illustrations in b , c and d were made using VESTA [34] . Full size image The highly correlated Kondo lattice compound UCu 5 is a heavy-fermion metal in which the coupling between its U 5f-electron spins and band electrons leads to a large electronic specific heat coefficient of γ~ 300 mJ mol K −2 , corresponding to an effective mass of its itinerant electrons nearly two orders of magnitude larger than that of a free electron [18] . Its magnetic U ions sit on a face-centred cubic (FCC) lattice and form a network of edge-sharing tetrahedra—a geometry conducive to magnetic frustration [1] ( Fig. 1b ). Curie–Weiss fits to the magnetic susceptibility give a Weiss temperature of θ W =−284 K, which reflects the strong anti-ferromagnetic interactions between magnetic ions [19] . Yet, UCu 5 orders magnetically at temperatures T ≪ θ W , first at T N =15.5 K, and then at T 2 =1.2 K, due in part to magnetic frustration [1] , [2] . Powder neutron diffraction experiments indicate that the anti-ferromagnetic order in both phases consists of localized U 5f-electron spins pointing along the crystal unit cell's <111> directions with ordering wave vectors symmetry related to q =<1/2,1/2,1/2> (refs 20 , 21 , 22 ), and the simplest magnetic order consistent with these data is the 1– q configuration shown in Fig. 1c with spins ferromagnetically aligned within (111) planes, but anti-ferromagnetically aligned with neighbouring (111) planes. The magnitude of q does not change when cooling through T 2 , despite clear signs of a phase transition in magnetization, resistivity and specific heat data, indicating that the transition is likely between single and multi- q states possessing the same | q |. In the absence of single crystals of UCu 5 , it is impossible to distinguish a multi-domain 1− q configuration from more complex multi- q variants using powder neutron diffraction measurements. Nevertheless, nuclear magnetic resonance experiments have revealed significant differences in the distribution of the local exchange field acting on the nuclei, consistent with a transition between distinct states with different numbers of ordered Fourier components of magnetization [23] . Here we report a strikingly large geometrical Hall effect below T 2 . On the basis of experimental results and theoretical analysis, we argue that the phase below T 2 possesses the 4– q non-coplanar anti-ferromagnetic order, illustrated in Fig. 1d , which causes a chirality-induced Berry phase in the itinerant electrons' wave functions and creates a large geometrical Hall effect that can be controlled by applying a relatively small magnetic field. Magnetic phase diagram and maximum in the hall resistivity The magnetic phase diagram for UCu 5 is shown in Fig. 2a , and we refer to the high- and low-temperature anti-ferromagnetic phases as M1 and M2, respectively. The phase diagram is constructed from M ( H ) data discussed below, as well as data shown in Supplementary Figs S1-S7 . M1 and M2 are phases possessing anti-ferromagnetic order, whereas PM is the paramagnetic phase. A Curie–Weiss fit to our susceptibility data is shown in Supplementary Fig. S2 and gives θ W =−238(2) K, which is much greater than T N and agrees with previous results [19] . 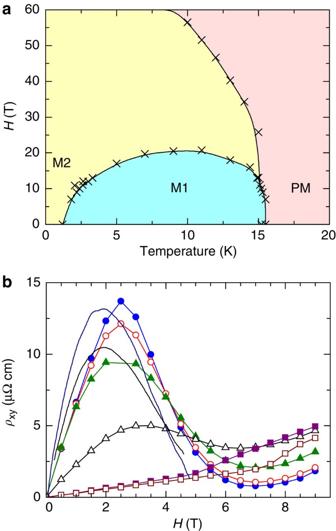Figure 2: Magnetic phase diagram and the Hall resistivity. (a) The phase diagram for UCu5. M1 and M2 are phases possessing the 1−qand 4−qanti-ferromagnetic order, respectively, whereas PM is the paramagnetic phase. The frustration-induced phase boundary between M1 and M2 at low fields agrees with earlier results35; however, we do not see the previously reported multiple phase transitions at higher fields, which is likely due to subtle differences between our samples and those in ref.35(see also ref.36andSupplementary Fig. S4). These differences are inconsequential to our conclusions. (b) The Hall resistivityρxyfor temperatures and fields spanning M1 and M2. Solid blue circles areT=0.05 K data, open red circles areT=0.2 K data, solid green triangles areT=0.5 K data, open black triangles areT=1.0 K data, solid purple squares areT=1.4 K data, and open wine squares areT=1.8 K data. In M1 (T=1.8 and 1.4 K),ρxy(H) is a simple function ofMandρxx, and can be described by the usual anomalous Hall effect mechanisms discussed in theSupplementary Methodssection of theSupplementary Information, but in M2 (T=0.05–1 K),ρxy(H) exhibits a peak nearH~2–2.5 T consistent with a geometrical Hall effect. Solid lines areT=0.65 K (blue) andT=0.85 K (black) data from a second separately prepared sample confirming the peak is intrinsic to M2. Figure 2: Magnetic phase diagram and the Hall resistivity. ( a ) The phase diagram for UCu 5 . M1 and M2 are phases possessing the 1− q and 4− q anti-ferromagnetic order, respectively, whereas PM is the paramagnetic phase. The frustration-induced phase boundary between M1 and M2 at low fields agrees with earlier results [35] ; however, we do not see the previously reported multiple phase transitions at higher fields, which is likely due to subtle differences between our samples and those in ref. 35 (see also ref. 36 and Supplementary Fig. S4 ). These differences are inconsequential to our conclusions. ( b ) The Hall resistivity ρ xy for temperatures and fields spanning M1 and M2. Solid blue circles are T =0.05 K data, open red circles are T =0.2 K data, solid green triangles are T =0.5 K data, open black triangles are T =1.0 K data, solid purple squares are T =1.4 K data, and open wine squares are T =1.8 K data. In M1 ( T =1.8 and 1.4 K), ρ xy ( H ) is a simple function of M and ρ xx , and can be described by the usual anomalous Hall effect mechanisms discussed in the Supplementary Methods section of the Supplementary Information , but in M2 ( T =0.05–1 K), ρ xy ( H ) exhibits a peak near H~ 2–2.5 T consistent with a geometrical Hall effect. Solid lines are T =0.65 K (blue) and T =0.85 K (black) data from a second separately prepared sample confirming the peak is intrinsic to M2. Full size image The Hall resistivity ρ xy ( H ) in both M1 and M2 is presented in Fig. 2b . Notably, in M2 ρ xy ( H ) has a pronounced peak near H~ 2-2.5 T, and the corresponding Hall conductivity σ xy =− ρ xy /( ρ xx 2 + ρ xy 2 ) is extremely large, exceeding 20% of the v =1 quantum Hall effect per atomic layer at H =2.5 T, which for free electrons with density of order one electron per unit cell would require H~ 10 3 T (ref. 24 ). In contrast, ρ xy ( H ) in M1 is a simple monotonic function of magnetization, consistent with standard spin–orbit coupling-dependent anomalous Hall effect mechanisms, such as skew scattering [9] , [10] ( Supplementary Fig. S7 ). The solid lines in Fig. 2b are data from a second separately prepared UCu 5 sample confirming the peak in ρ xy ( H ) is intrinsic to M2. Magnetization and magnetoresistance To examine the possible mechanisms responsible for the observed maximum in the low-temperature Hall resistance, the field- and temperature-dependent Hall responses should be compared with M ( H ) and ρ xx ( H ) for temperatures and fields spanning M1 and M2. 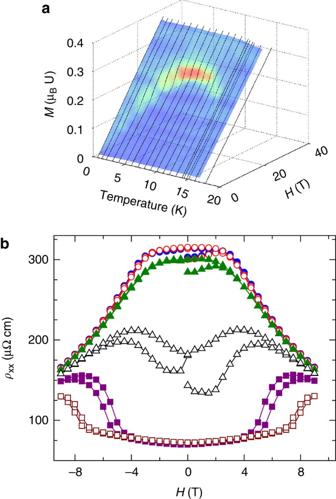Figure 3: Magnetization and longitudinal resistivity for temperatures and fields spanning M1 and M2. (a) Image plot of the field dependence of the magnetizationMfor various temperatures. Different colours indicate the slope dM/dH.M(H) is linear in both M1 and M2, with a change of slope occurring at the phase boundary. (b) The field dependence of the longitudinal resistivityρxxfor various temperatures. Solid blue circles areT=0.05 K data, open red circles areT=0.2 K data, solid green triangles areT=0.5 K data, open black triangles areT=1.0 K data, solid purple squares areT=1.4 K data, and open wine squares areT=1.8 K data. ForT<1 K,ρxx(H) is nearly constant up toH~2.5 T, but forT=1.8 and 1.4 K, hysteresis occurs atH~7 and 4 T, respectively, as the M1–M2 boundary is crossed. AtT=1 K, hysteresis occurs over most of the field range, consistent with the steep-phase boundary. Figure 3a is an image plot of M ( H ) in which different colours correspond to d M /d H and highlight the M1–M2 phase boundary. In M1, M ( H ) is linear for fields up to the M1–M2 phase boundary where there is a step increase. After the step, M ( H ) continues linearly in M2, but with a larger slope, and M ( H ) is linear in M2 for all temperatures and fields measured. Figure 3b shows that at T =1.4 and 1.8 K ρ xx ( H ) exhibits a positive magnetoresistance in M1, with hysteresis occurring at the M1–M2 phase boundary. Once a high-enough field is reached to cross into M2, ρ xx ( H ) has negative magnetoresistance in agreement with T =0.05–0.2 K data. T =1 K data show large hysteresis near the M1–M2 boundary, which is consistent with the previously reported sharp temperature–hysteretic peak at T 2 in specific heat indicative of a first order transition [18] . ρ xx ( H ) in M2 shows a difference between virgin and field-cycled curves, but no other hysteresis. Figure 3: Magnetization and longitudinal resistivity for temperatures and fields spanning M1 and M2. ( a ) Image plot of the field dependence of the magnetization M for various temperatures. Different colours indicate the slope d M /d H . M ( H ) is linear in both M1 and M2, with a change of slope occurring at the phase boundary. ( b ) The field dependence of the longitudinal resistivity ρ xx for various temperatures. Solid blue circles are T =0.05 K data, open red circles are T =0.2 K data, solid green triangles are T =0.5 K data, open black triangles are T =1.0 K data, solid purple squares are T =1.4 K data, and open wine squares are T =1.8 K data. For T <1 K, ρ xx ( H ) is nearly constant up to H~ 2.5 T, but for T =1.8 and 1.4 K, hysteresis occurs at H ~7 and 4 T, respectively, as the M1–M2 boundary is crossed. At T =1 K, hysteresis occurs over most of the field range, consistent with the steep-phase boundary. Full size image Ruling out conventional anomalous Hall effect mechanisms The highly unconventional peak in ρ xy ( H ) in M2 contrasts with the featureless behaviour of both ρ xx ( H ) and M ( H ). At T <0.5 K, Fig. 3b shows that ρ xx ( H ) is almost constant up to H =3T, even as a peak in ρ xy ( H ) is reached at H~ 2–2.5 T. Similarly, in M2, M ( H ) is linear in H and does not show any anomalies around H~ 2–2.5 T. Therefore, in contrast to ρ xy ( H ) in M1, the unusual behaviour of ρ xy ( H ) in M2 is not dominated by the standard anomalous Hall effect due to the spin–orbit interaction. The differences in behaviour between ρ xy ( H ) in the M1 and M2 phases is particularly clear in the derivative d σ xy /d M ( Supplementary Fig. S8a ). In the low-field region of M2, the behaviour of σ xy is highly unconventional with d σ xy /d M changing sign with increasing H , and Supplementary Fig. S8b shows that the maximum in ρ xy ( H ) cannot be fit assuming skew scattering alone. This is the regime in which a geometrical Hall effect due to the acquired chirality-induced Berry phase dominates. To demonstrate how a chirality-induced geometrical Hall effect arises due to the non-coplanar 4− q magnetic order, we analyse the properties of UCu 5 within the Kondo lattice model (KLM) for an FCC lattice: where σ δ are the Pauli matrices, c is the annihilation operator for the itinerant electrons, < i , j > indicates nearest-neighbour U sites, t is the hopping matrix element for the current of itinerant electrons, and S δ is the component of the U spin in the δ direction. The dynamical Kondo coupling J K gives the coupling strength between itinerant electrons and U spins, and is the origin of the large effective mass [18] . Here, we will concentrate on the magnetically ordered phases and assume that local moments are classical. Using a variational calculation [24] , we find that depending on J K and the carrier density of the current, n , both the 1− q and 4− q states, among others, can be stabilized at T =0. A typical parameter set to stabilize 4− q order is J K / t =3.5 with n =0.3 electrons per site. It is possible to study the thermodynamic phase transitions of the KLM directly [24] , but it is very computationally intensive. Therefore, for finite temperature calculations, we use a related classical spin model which gives the same result as the KLM at T =0, Here, S is the spin of Uranium, J 1 and J 2 are the anti-ferromagnetic exchange coupling strengths between nearest and next-nearest neighbours, respectively, K is the nearest-neighbour biquadratic exchange strength, and the final term allows coupling to an applied magnetic field. For 2 J 2 > J 1 and K =0 the model yields a continuum of ground states due to magnetic frustration. Single spin-flip Monte-Carlo simulations using J 1 =1.5, J 2 =1 and K =0.01, which give the experimentally observed ratio of T N / T 2 , yield the H =0 specific heat curve shown in Fig. 4a . The simulations reproduce the two-phase transitions, with the lower-temperature phase possessing the 4− q order and the higher-temperature phase possessing the 1− q order (within the framework of these simulations, the transitions at T 2 and T N appear to be first and second order, respectively, which is consistent with experiments; the order of the transitions, however, has not yet been confirmed with complete certainty due to computational limitations). The transition between M2 and M1 is driven by thermal fluctuations favouring the 1− q state, because the order-by-disorder mechanism stabilizes coplanar magnetic order at finite temperature for a frustrated FCC lattice [25] , [26] . We note that the analysis of the NMR data in ref. 23 gives M1 as the 4− q state and M2 as the 1− q state. However, the 4− q state is expected to be more energetically favourable than the 1− q state in Kondo-lattice systems. Indeed, a highly frustrated insulator Gd 2 Ti 2 O 7 has been shown to have a 4− q ground state and a 1− q state at higher temperatures [26] . This trend also is consistent with general theoretical arguments that thermal fluctuations tend to stabilize the simpler magnetic configuration [25] . Moreover, ρ xx ( T ) data for Lu 0.02 U 0.98 Cu 5 shown in Supplementary Fig. S9 show an increase in T 2 with non-magnetic dilution, which is also consistent with order-by-disorder. 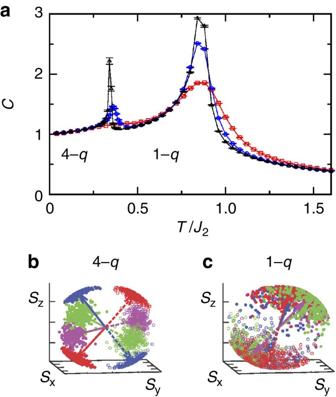Figure 4: Monte-Carlo simulation results reproducing the experimentally observed magnetic phase transitions. (a) The calculated heat capacityCversus the reduced temperatureT/J2usingJ1=1.5,J2=1, andK=0.01. The different curves correspond to different lattice sizes (L=4: red squares;L=6: blue circles;L=8: black triangles). (b) A snapshot of the spin structure taken during the Monte-Carlo simulations showing that 4−qanti-ferromagnetic order exists below the lower temperature phase transition. (c) A snapshot of the spin structure taken during the Monte-Carlo simulations showing that 1−qanti-ferromagnetic order exists between the lower and higher temperature phase transitions. Figure 4b and c show snapshots taken during the simulations of the spin configurations in the 4− q and 1− q phases, respectively. In the KLM, we have treated the spins classically and have not assumed any spin–orbit coupling, which is the key ingredient in most anomalous Hall-effect theories, and has been shown to be important in explaining the Hall effect in Pr 2 Ir 2 O 7 and Nd 2 Mo 2 O 7 (ref. 27 ). Figure 4: Monte-Carlo simulation results reproducing the experimentally observed magnetic phase transitions. ( a ) The calculated heat capacity C versus the reduced temperature T / J 2 using J 1 =1.5, J 2 =1, and K =0.01. The different curves correspond to different lattice sizes ( L =4: red squares; L =6: blue circles; L =8: black triangles). ( b ) A snapshot of the spin structure taken during the Monte-Carlo simulations showing that 4− q anti-ferromagnetic order exists below the lower temperature phase transition. ( c ) A snapshot of the spin structure taken during the Monte-Carlo simulations showing that 1− q anti-ferromagnetic order exists between the lower and higher temperature phase transitions. Full size image Unlike spins, the scalar-spin chirality does not couple directly to a magnetic field and is invariant to the rigid rotation of all the spins that can be induced by a rotation of an external magnetic field. Therefore, it may appear that the Hall effect attributable to the scalar spin chirality must average to zero for polycrystalline samples. The presence of itinerant electrons prevents this, because electrons moving in a chiral texture acquire orbital magnetization [28] that directly couples to the magnetic field. For the experimental values of σ xy calculated from data in Fig. 2b , the orbital magnetization per unit cell is estimated to be ~ 10 −2 μ B ; therefore, at T ~1 K, a magnetic field of only 1 Tesla should be sufficient to align even small domains containing 100 unit cells. Thus, the acquired orbital magnetization can produce an experimental signature of a large geometrical Hall effect, even in polycrystalline samples. Given this coupling between the orbital magnetization and magnetic field, we calculate σ xy ( H ) at T =0 by first choosing among the multiple energetically equivalent ground states of equation (2) with different values of the scalar spin chirality χ 111 projected on to the [111] direction, which for the purpose of our calculations we assume to be parallel to H . We then select the state with the largest χ 111 to give us an initial spin configuration as this state will be favoured by the coupling between the orbital magnetization and H . Fig. 5a shows χ 111 ( H ) and examples of the spin configurations for different H . Next, we substitute the determined spin configurations into equation (1) and use the Kubo formula [29] to calculate the chirality-induced Berry phase contribution to σ xy ( H ). Fig. 5b and c show the measured and calculated σ xy ( H ) curves, respectively. Remarkably, both curves show a local minimum as a function of magnetic field and have comparable magnitudes, despite the simplistic way in which we have chosen the Hamiltonian parameters. Though qualitative in nature, these calculations demonstrate that the magnetic field distortion of the 4− q magnetic order can induce an extremely strong response in the Hall conductivity, comparable to experimental results, and illustrate the principle of generating large geometric Hall responses with a field due to a non-coplanar spin texture without assuming any material-specific spin–orbit interaction. 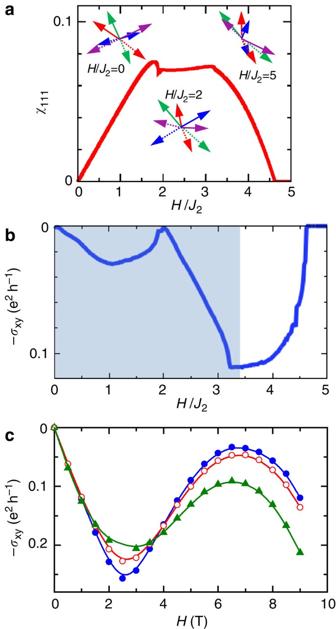Figure 5: Field-controlled geometrical Hall effect due to the frustration-induced 4−qmagnetic order. (a) The scalar spin chiralityχ111atT=0 as a function of the external magnetic field,H. Examples of spin configurations obtained by mean field analysis of the Hamiltonian (2) corresponding to different values ofχ111are also shown. (b) The calculatedT=0 Hall conductivityσxydue to the geometrical Hall effect as a function of magnetic fieldHin the frustration-induced 4−qmagnetically ordered state (J1=1.5,J2=1,K=0.01,JK/t=3.5,n=0.3). (c) The experimentally observed Hall conductivity as a function ofH. Solid blue circles areT=0.05 K data, open red circles areT=0.2 K data, and solid green triangles areT=0.5 K data. In the shaded region ofb, the calculation reproduces the minimum in the experimental data shown incalong with the rise of |σxy| at higher fields. The calculated values ofσxy(H) arise solely from the acquired chirality-induced Berry phase and do not include material specific spin–orbit effects. Similar calculations assuming 1−qmagnetic order do not yield a finite chirality-induced Berry phase contribution toσxy(H). Figure 5: Field-controlled geometrical Hall effect due to the frustration-induced 4− q magnetic order. ( a ) The scalar spin chirality χ 111 at T =0 as a function of the external magnetic field, H . Examples of spin configurations obtained by mean field analysis of the Hamiltonian (2) corresponding to different values of χ 111 are also shown. ( b ) The calculated T =0 Hall conductivity σ xy due to the geometrical Hall effect as a function of magnetic field H in the frustration-induced 4− q magnetically ordered state ( J 1 =1.5, J 2 =1, K =0.01, J K / t =3.5, n =0.3). ( c ) The experimentally observed Hall conductivity as a function of H . Solid blue circles are T =0.05 K data, open red circles are T =0.2 K data, and solid green triangles are T =0.5 K data. In the shaded region of b , the calculation reproduces the minimum in the experimental data shown in c along with the rise of | σ xy | at higher fields. The calculated values of σ xy ( H ) arise solely from the acquired chirality-induced Berry phase and do not include material specific spin–orbit effects. Similar calculations assuming 1− q magnetic order do not yield a finite chirality-induced Berry phase contribution to σ xy ( H ). Full size image These results strongly suggest that the peak in ρ xy ( H ) in the M2 phase is due to a chirality-induced Berry phase caused by the frustration-created spin texture. Although previous works on Nd 2 Mo 2 O 7 and Pr 2 Ir 2 O 7 have argued for observation of such a geometrical Hall effect [12] , [13] , it has been contested that in these cases, the Hall effect primarily stems from the magnetic Mo or Ir ions and is due to the d -orbital angular momentum induced by the spin–orbit interaction rather than being induced by the non-coplanar spin textures of the Nd or Pr [27] . In our case, Cu is not magnetic and the chirality-induced Berry phase is due to magnetic exchange between f and d electrons. Also, the Berry phase due to spin–orbital effects in the electronic band structure should be insensitive to small amounts of disorder. As we show in Supplementary Figs S9 and S10 , and discuss in the Supplementary Methods section, Hall measurements on UCu 5− x M x , with M =Ag or Au and x =0.01, 0.03 (that is, 0.2 and 0.6% substitution) and U 1− x Lu x Cu 5 , x =0.02 show that the peak in ρ xy ( H ) is suppressed by small, nominally isoelectronic substitutions. These experiments rule against a notable contribution to the Berry phase from the spin–orbit induced momentum–space monopoles [9] and demonstrate that the 4− q order in UCu 5 is necessary for the observed geometrical Hall effect. Finally, a chirality-induced Berry phase effect also has been proposed to explain σ xy in MnSi (refs 30 , 31 ) and MnGe [32] ; however, in these cases, the induced Hall effect is orders of magnitude weaker than in UCu 5 due to the very smooth nature of the Skyrmion [33] textures. We have shown that a tunable, unusually large Hall conductivity, equivalent to the presence of an effective magnetic field of ~ 10 3 T, arises in UCu 5 , and that the chirality-induced Berry phase due to frustration-induced non-coplanar 4− q anti-ferromagnetic order creates this large geometrical Hall effect. These results provide an example of the possible exotic transport properties resulting from magnetic frustration in highly correlated metals, whereas illustrating the opportunities afforded by pursuing studies on other frustrated metals. In particular, control of the geometrical Hall effect by a small magnetic field shows that frustration can be an important tuning parameter, allowing for the tailoring of specific properties and states of correlated matter. Sample synthesis Polycrystalline samples of UCu 5.1 and UCu 5.05 were prepared by arc melting on a water-cooled Cu hearth under an Ar atmosphere, followed by annealing under vacuum (10 −4 Torr) at 800 or 850 °C for 1–3 weeks. Samples were determined to be single phase by X-ray diffraction, and we confirmed that both UCu 5.1 and UCu 5.05 share the same field-temperature phase diagram. Hence, for simplicity, we refer to both samples as UCu 5 . The UCu 5− x M x , M =Ag, Au, x =0.01, 0.03, and U 0.98 Lu 0.02 Cu 5 samples were made in a similar fashion. Magnetization measurements Magnetization measurements were made in a Quantum Design Superconducting Quantum Interference Device magnetometer, in a dilution refrigerator utilizing either a capacitance-based Faraday or torque magnetometer, and in pulsed magnetic fields using a compensated coil-extraction magnetometer. Resistivity measurements Four-wire resistivity measurements of the longitudinal resistivity and Hall resistivity were performed on thin rectangular samples using a Linear Research LR-700 ac resistance bridge, and the samples were cooled and exposed to a magnetic field in a Quantum Design Physical Property Measurement System or a dilution refrigerator with an incorporated magnet. Pt leads were attached to the samples by either spot welding or by applying silver paint. Longitudinal contributions to the Hall resistivity were cancelled by making measurements in both positive and negative fields. High-field measurements were made at the National High Magnetic Field Laboratories in Tallahassee and Los Alamos. How to cite this article: Ueland, B.G. et al . Controllable chirality-induced geometrical Hall effect in a frustrated highly correlated metal. Nat. Commun. 3:1067 doi: 10.1038/ncomms2075 (2012).